A Snail1/Notch1 signalling axis controls embryonic vascular development Notch1-Delta-like 4 (Dll4) signalling controls vascular development by regulating endothelial cell (EC) targets that modulate vessel wall remodelling and arterial–venous specification. The molecular effectors that modulate Notch signalling during vascular development remain largely undefined. Here we demonstrate that the transcriptional repressor, Snail1, acts as a VEGF-induced regulator of Notch1 signalling and Dll4 expression. EC-specific Snail1 loss-of-function conditional knockout mice die in utero with defects in vessel wall remodelling in association with losses in mural cell investment and disruptions in arterial–venous specification. Snail1 loss-of-function conditional knockout embryos further display upregulated Notch1 signalling and Dll4 expression that is partially reversed by inhibiting γ-secretase activity in vivo with Dll4 identified as a direct target of Snail1-mediated transcriptional repression. These results document a Snail1-Dll4/Notch1 axis that controls embryonic vascular development. The evolutionarily conserved Notch signalling pathway plays critical roles in controlling multiple aspects of vascular development and endothelial cell (EC) function, ranging from proliferation, motility and lumen formation to vessel stability and cell fate determination [1] , [2] . In vertebrates, the Notch signalling pathway consists of four Notch family receptors (Notch1–Notch4) and five Notch ligands ((Jagged1, Jagged2, Delta-like (Dll) 1, Dll3 and Dll4)) [2] . Receptor-ligand interactions between neighbouring cells initiates the proteolytic cleavage of the Notch receptor extracellular domain, the γ-secretase-dependent release of the Notch intracellular domain, and its subsequent translocation to the nucleus where it associates with the DNA-binding protein, RBPJK/CBF1/Su(H), as well as a co-activator of the Mastermind-like family, thereby triggering the transcription of downstream target genes, including Hey/Hes family members [2] . EC-specific deletion or overexpression of key components of the Notch signalling pathway, for example, Notch1, its transcriptionally active intracellular form (N1ICD) or Dll4, impinges on the normal development of the embryonic vasculature and results in early embryonic lethality [3] , [4] , [5] . Recent studies suggest that vascular endothelial growth factor (VEGF), ETS factors, Sox and Notch regulate Dll4 expression in complex cascades that may be further impacted by the canonical Wnt pathway [1] , [6] , [7] , [8] , [9] . However, despite the fact that even subtle changes in Dll4 expression impair vascular development [2] , [4] , [10] , [11] , [12] , the regulatory systems that fine-tune Dll4/Notch signalling during the development of the embryonic vasculature in vivo remain largely undefined. The zinc-finger transcriptional repressor, Snail1, has been shown to play an essential role in the induction of epithelial–mesenchymal transition (EMT) and gastrulation in the developing mouse embryo [13] . Mouse embryos homozygous for a Snail1-null mutation (Snail1 −/− embryos) display defects in mesoderm formation and die shortly after embryonic day (E) 7.5 (ref. 14 ). Recently, Gridley and colleagues [15] , [16] reported that the epiblast-specific deletion of Snail1 at later stages in mouse embryonic development is permissive for normal gastrulation, but results in defective left–right asymmetry determination and cardiovascular development. However, as all embryonic tissues were rendered Snail1 deficient in these studies, the possibility that Snail1 functions in an EC-autonomous fashion in vivo remains unexplored. Here we report that EC-specific Snail1 loss-of-function (LOF) conditional knockout (KO) mice display an early embryonic lethal phenotype with marked defects in vascular remodelling, morphogenesis and arterial–vein specification. Unexpectedly, the observed changes in vascular development phenocopy a subset of the defects commonly associated with upregulated Dll4/Notch1 signalling [4] , [5] , [6] . Indeed, we now identify Snail1 as a VEGF-induced, cis -acting, negative feedback regulator of Dll4 and Notch1 expression in vitro and in vivo . These studies characterize a novel, EMT-independent function of Snail1, whereby the transcription factor as a required regulator of the Notch signalling cascade that controls vascular development during embryogenesis. EC-specific Snail1 deletion leads to embryonic lethality To interrogate a potential role for Snail1 during embryonic vascular development, conditional Snail1 fl/fl mice [17] were crossed with a Tie2 -Cre transgenic line, thereby targeting Cre recombinase in ECs as well as haematopoietic stem cells [18] . Under these conditions, no viable pups expressing Snail1 fl/fl ; Tie2 -Cre + (that is, Snail1 LOF mutants) were born ( Fig. 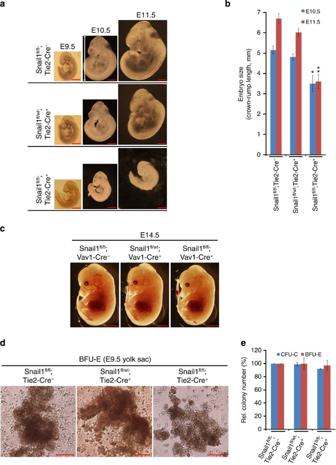Figure 1: Endothelial-specific deletion of Snail1 induces embryonic lethality. (a) Gross examination of whole embryos at the indicated stages of development. Note the significantly reduced size ofSnail1fl/fl;Tie2-Cre+embryos at E10.5 and E11.5. Scale bar, 1 mm. (b) Quantification of embryo size as indicated by crown-rump length (shown ina) (n=4 in each group). Data are presented as mean±s.e.m. *P<0.05 and **P<0.01 (analysis of variance (ANOVA) test). (c) Gross examination of whole embryos fromVav1-Cre crosses at E14.5. No differences were observed betweenSnail1fl/fl;Vav1-Cre+mutants and their control littermates in size, stage or overall appearance. Scale bars, 2 mm. (d,e)In vitrodifferentiation analysis of yolk sac haematopoietic cells derived from E9.5Snail1fl/fl;Tie2-Cre+mutants and their control littermates. Representative photomicrographs of BFU-E colonies 7 days after plating are shown at left (d). Quantification of CFU-E and BFU-E colonies from yolk sacs (n=3 in each group) is shown to the right (e). Data are presented as mean±s.e.m. Not significant, ANOVA. Scale bars, 50 μm. 1a and Table 1 ). In timed matings, Snail1 LOF embryos are morphologically indistinguishable from control embryos (that is, littermates expressing Snail1 fl/wt ; Tie2 -Cre + or Snail1 fl/fl ; Tie2 -Cre − ) up to E9.5 ( Fig. 1a ). However, by E10.5 and E11.5, Snail1 LOF mutant embryo size (crown-rump length) is decreased by 32 and 47%, respectively, as compared with their control littermates ( Fig. 1b ). Furthermore, ~50 and 100% of Snail1 LOF embryos die at E11.5 or 12.5, respectively ( Table 1 ), demonstrating that the Tie2 -Cre-driven deletion of Snail1 dramatically impacts early embryonic development. Figure 1: Endothelial-specific deletion of Snail1 induces embryonic lethality. ( a ) Gross examination of whole embryos at the indicated stages of development. Note the significantly reduced size of Snail1 fl/fl ; Tie2 -Cre + embryos at E10.5 and E11.5. Scale bar, 1 mm. ( b ) Quantification of embryo size as indicated by crown-rump length (shown in a ) ( n =4 in each group). Data are presented as mean±s.e.m. * P <0.05 and ** P <0.01 (analysis of variance (ANOVA) test). ( c ) Gross examination of whole embryos from Vav1 -Cre crosses at E14.5. No differences were observed between Snail1 fl/fl ; Vav1 -Cre + mutants and their control littermates in size, stage or overall appearance. Scale bars, 2 mm. ( d , e ) In vitro differentiation analysis of yolk sac haematopoietic cells derived from E9.5 Snail1 fl/fl ; Tie2 -Cre + mutants and their control littermates. Representative photomicrographs of BFU-E colonies 7 days after plating are shown at left ( d ). Quantification of CFU-E and BFU-E colonies from yolk sacs ( n =3 in each group) is shown to the right ( e ). Data are presented as mean±s.e.m. Not significant, ANOVA. Scale bars, 50 μm. Full size image Table 1 Viable progeny from Snail1 fl/fl mice intercrossed with Snail1 fl/wt ; Tie2 -Cre + mice as a function of age. Full size table To further specify the cell lineage that contributes to Snail1 LOF-induced embryonic lethality, conditional Snail1 fl/fl mice were crossed with a Vav1 -Cre line that drives Cre recombinase expression specifically in haematopoietic cells during definitive haematopoiesis [19] . In marked contrast to the Tie2 -Cre + mice, analysis of embryos at E14.5, E17.5 or postnatal day 1 (P1) demonstrated no differences in viability or gross morphology between Snail1 fl/fl ;Vav1 -Cre + mutants and control littermates expressing Snail1 fl/wt ; Vav1 -Cre + or Snail1 fl/fl ; Vav1 -Cre − ( Fig. 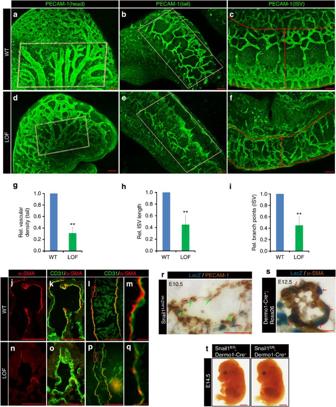Figure 2: Endothelial-specific deletion of Snail1 derails vascular development. Whole-mount PECAM-1 immunofluorescent staining of E10.5 WT (a–c) and Snail1 LOF (d–f) embryos. Defective remodelling and branching are highlighted in the cephalic (rectangled area inaandd), tail (rectangled area inbande) and ISVs (area demarcated by dotted lines incandfwith ISV width of field marked by the double-headed arrows). Scale bar, 100 μm. (g–i) Quantification of relative vascular density in tail (PECAM-1-positive vessel area in rectangle box;g) vessels as well as vessel length (h) and branch points (defined as the junction point of three vessels;i) of ISV in WT and Snail1 LOF embryos (n=4 in each group). Data are presented as mean±s.e.m. **P<0.01, Student’sttest. Cross-sections (j,k,n,o) and sagittal sections (l,m,p,q) obtained from E10.5 WT (j–m) and Snail1 LOF (n–q) embryos were stained with anti-PECAM and anti-α-SMA antibodies to detect ECs and vascular smooth muscle cells, respectively. Boxed areas inlandpare shown at higher magnification inmandq, respectively. The arteries in WT embryos are surrounded by α-SMA-positive cells, whereas arteries in LOF embryos recruited few α-SMA-positive cells. Scale bar, 50 μm (j,k,n,o); 100 μm (l,p); 10 μm (m,q). (r) Cross-sections from E10.5 Snail1LacZ/wtembryos were stained with X-Gal/lacZ followed by PECAM-1 immunohistochemical staining. Green or red arrows denote the Snail1-positive ECs and perivascular cells, respectively. Scale bar, 50 μm. (s) Cross-sections from E12.5 ROSA26;Dermo1-Cre+embryos were stained with X-Gal/lacZ followed by α-SMA immunohistochemical staining. Red arrows mark dual-positive perivascular cells. Scale bar, 50 μm. (t) Gross examination of whole embryos fromDermo1-Cre crosses at E14.5. No differences were observed betweenSnail1fl/fl;Dermo1-Cre+mutants and their control littermates in size, stage or overall appearance. Scale bar, 2 mm. 1c and Table 2 ), indicating that Snail1 deletion confined to haematopoietic cells alone does not phenocopy Snail1 LOF mutants. As yolk sac-derived blood islands serve as the sole source of primitive haematopoietic cell production up to E9.5 (a stage before Vav1 -Cre is expressed) [20] , we further used haematopoietic colony-forming assays to assess the potential impact of Tie2 -Cre-mediated Snail1 deletion on early stages of haematopoiesis. However, in vitro differentiation of yolk sac haematopoietic progenitor cells derived from E9.5 Snail1 LOF mutants and control littermates demonstrates comparable erythroid colony formation (CFU-E and BFU-E) ( Fig. 1d,e ). Taken together, these data support a model wherein the loss of Snail1 expression in the endothelial compartment is incompatible with early embryonic development. Table 2 Viable progeny from Snail1 fl/fl mice intercrossed with Snail1 fl/wt ; Vav1 -Cre + mice as a function of age. Full size table Snail1 LOF mutant embryos display vascular deficits At E10.5, Snail1 LOF embryos are smaller in size with associated defects in the patterning of several regions of the vascular tree despite similar somite numbers (35±3 somites in wild type (WT) versus 33±2 somites in LOF; n =4) ( Fig. 2a–f ). Cranial blood vessels fail to undergo the remodelling events that normally lead to the generation of larger caliber vessels (compare Fig. 2a,d boxed areas). Vascularization of the tail is also impaired in Snail1 LOF embryos with the formation of truncated and disorganized networks ( Fig. 2b,e,g ). Intersomitic vessels (ISV), formed through angiogenic sprouting [21] , are present in the Snail1 LOF mutant embryos, but are unable to organize or fully infiltrate the somites (compare Fig. 2c,f ), displaying significant decreases in ISV length and branch points ( Fig. 2h,i ). Although Snail1 can exert anti-apoptotic effects in expressing cell populations [22] , no differences in the number of TUNEL (TdT-mediated dUTP nick end labelling)-positive ECs within the dorsal aorta (DA) or surrounding vessels are observed between WT and Snail1 LOF embryos ( Supplementary Fig. 1a–c ). Figure 2: Endothelial-specific deletion of Snail1 derails vascular development. Whole-mount PECAM-1 immunofluorescent staining of E10.5 WT ( a – c ) and Snail1 LOF ( d – f ) embryos. Defective remodelling and branching are highlighted in the cephalic (rectangled area in a and d ), tail (rectangled area in b and e ) and ISVs (area demarcated by dotted lines in c and f with ISV width of field marked by the double-headed arrows). Scale bar, 100 μm. ( g – i ) Quantification of relative vascular density in tail (PECAM-1-positive vessel area in rectangle box; g ) vessels as well as vessel length ( h ) and branch points (defined as the junction point of three vessels; i ) of ISV in WT and Snail1 LOF embryos ( n =4 in each group). Data are presented as mean±s.e.m. ** P <0.01, Student’s t test. Cross-sections ( j , k , n , o ) and sagittal sections ( l , m , p , q ) obtained from E10.5 WT ( j – m ) and Snail1 LOF ( n – q ) embryos were stained with anti-PECAM and anti-α-SMA antibodies to detect ECs and vascular smooth muscle cells, respectively. Boxed areas in l and p are shown at higher magnification in m and q , respectively. The arteries in WT embryos are surrounded by α-SMA-positive cells, whereas arteries in LOF embryos recruited few α-SMA-positive cells. Scale bar, 50 μm ( j , k , n , o ); 100 μm ( l , p ); 10 μm ( m , q ). ( r ) Cross-sections from E10.5 Snail1 LacZ/wt embryos were stained with X-Gal/lacZ followed by PECAM-1 immunohistochemical staining. Green or red arrows denote the Snail1-positive ECs and perivascular cells, respectively. Scale bar, 50 μm. ( s ) Cross-sections from E12.5 ROSA26; Dermo1 -Cre + embryos were stained with X-Gal/lacZ followed by α-SMA immunohistochemical staining. Red arrows mark dual-positive perivascular cells. Scale bar, 50 μm. ( t ) Gross examination of whole embryos from Dermo1 -Cre crosses at E14.5. No differences were observed between Snail1 fl/fl ; Dermo1 -Cre + mutants and their control littermates in size, stage or overall appearance. Scale bar, 2 mm. Full size image Independent of vascular patterning defects, immunostaining for α-smooth muscle actin (α-SMA), a marker for vascular smooth muscle cells, demonstrates that although the DA of WT E10.5 embryos are surrounded by α-SMA-positive cells, arteries in Snail1 LOF embryos fail to develop well-developed, α-SMA-positive mural coats ( Fig. 2j–q ). Interestingly, using Snail1 LacZ/wt mice [23] , β-galactosidase reporter activity is not only detected in PECAM-1-positive ECs within the DA, vitelline artery and cardinal vein, but also in PECAM-1-negative, perivascular cells surrounding arterial beds ( Fig. 2r and Supplementary Fig. 2a–j ). To determine whether perivascular Snail1 is also required during embryonic development, Snail1 fl/fl mice were next crossed with a Dermo1 -Cre transgenic line [24] , thereby targeting Cre recombinase throughout the mesoderm, including the mural cell compartment as assessed in Dermo1-Cre + ;Rosa26 crosses [25] , [26] ( Fig. 2s ). However, analyses of embryos at E14.5 or P1 demonstrated no differences in viability or gross morphology between Snail1 fl/fl ; Dermo1 -Cre + mutants and control littermates expressing Snail1 fl/fl ; Dermo1 -Cre − ( Fig. 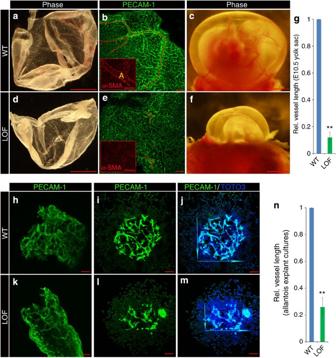Figure 3: EC Snail1 drives vascular remodelling in extra-embryonic tissues. Gross examination of yolk sacs dissected from E10.5 WT (a) and Snail1 LOF (d) embryos. Scale bar, 2 mm. Whole-mount PECAM-1 staining of yolk sac dissected from E10.5 WT (b) and Snail1 LOF (e) embryos. Insets, representative images of whole-mount α-SMA staining. Red lines mark continuous vessels with a diameter⩾20 μm. Scale bar, 100 μm. Gross examination of WT (c) and Snail1 LOF (f) embryos with yolk sac at E11.5. Note the absence of vascular structures in the LOF mutant yolk sacs. Scale bar, 2 mm. (g) Quantification of relative vessel (diameter⩾20 μm) length in yolk sacs from E10.5 WT (b) and Snail1 LOF (e) embryos (n=4 each). Data are presented as mean±s.e.m. **P<0.01, Student’sttest. Whole-mount PECAM-1 staining of allantois explants dissected from E8.25 WT (h–j) and Snail1 LOF (k–m) embryos. At pre-culture (h,k), vascularization of allantois explants derived from WT and Snail1 LOF embryos were comparable, whereas at 24 h post culture, the Snail1 LOF embryo explants display marked defects in their ability to generate vascular structures (i,j,l,m). Cell nuclei were stained with TOTO3 (blue). Scale bar, 100 μm. (n) Quantification of relative vessel length in the WT and Snail1 LOF explant cultures (n=5 in each group). Data are presented as mean±s.e.m. **P<0.01, Student’st-test. 2t and Table 3 ), indicating that Snail1 expression in mural cell populations does not play a major role during embryonic vascular development. Table 3 Viable progeny from Snail1 fl/fl mice intercrossed with Snail1 fl/wt ; Dermo1 -Cre + mice as a function of age. Full size table Outside the embryo proper, yolk sacs in Snail1 LOF mutants at E10.5 display multiple vascular defects, including gross reductions in the number of perfused blood vessels in combination with marked tissue pallor (compare Fig. 3a,d ). Strikingly, PECAM-1 whole-mount staining reveals the severely defective remodelling of the primary vascular plexus into both hierarchical and branched vessels in the Snail1 LOF yolk sacs (compare Fig. 3b,e ). Further, α-SMA staining demonstrates that although arteries of WT yolk sacs are surrounded by α-SMA-positive cells, vessels in Snail1 LOF yolk sacs fail to develop α-SMA-positive mural coats (compare insets in Fig. 3b,e ). Quantification of vascularization (that is, small and large vessels arising from the primordial vascular plexus) highlights the almost complete loss of vessel remodelling in Snail1 LOF mutants at E10.5 ( Fig. 3g ). The vascular phenotype of mutants further progressed until E11.5, at which time ~50% of embryos are necrotic with no intact vascular structures remaining (compare Fig. 3c,f ). Vascular defects are also observed in the labyrinthine layer of the placenta, a tissue that is essential for gas and nutrient exchange during gestation [27] ( Supplementary Fig. 3a–f ). Under normal conditions, the allantois attaches to the chorionic plate (the initial step in the formation of a functional placenta), which is followed by vascular invasion of the labyrinthine layer [27] . In Snail1 LOF mutants, however, although the chorionic plate and trophoblast giant cells appear normal in structure and number, the labyrinthine layer is reduced in thickness and vascularization relative to WT littermates ( Supplementary Fig. 3a–f ). Further, in Snail1 LOF mutants, the number of fetal blood vessels that invade and interdigitate into the labyrinthine layer is reduced markedly ( Supplementary Fig. 3a–f ). Figure 3: EC Snail1 drives vascular remodelling in extra-embryonic tissues. Gross examination of yolk sacs dissected from E10.5 WT ( a ) and Snail1 LOF ( d ) embryos. Scale bar, 2 mm. Whole-mount PECAM-1 staining of yolk sac dissected from E10.5 WT ( b ) and Snail1 LOF ( e ) embryos. Insets, representative images of whole-mount α-SMA staining. Red lines mark continuous vessels with a diameter ⩾ 20 μm. Scale bar, 100 μm. Gross examination of WT ( c ) and Snail1 LOF ( f ) embryos with yolk sac at E11.5. Note the absence of vascular structures in the LOF mutant yolk sacs. Scale bar, 2 mm. ( g ) Quantification of relative vessel (diameter ⩾ 20 μm) length in yolk sacs from E10.5 WT ( b ) and Snail1 LOF ( e ) embryos ( n =4 each). Data are presented as mean±s.e.m. ** P <0.01, Student’s t test. Whole-mount PECAM-1 staining of allantois explants dissected from E8.25 WT ( h – j ) and Snail1 LOF ( k – m ) embryos. At pre-culture ( h , k ), vascularization of allantois explants derived from WT and Snail1 LOF embryos were comparable, whereas at 24 h post culture, the Snail1 LOF embryo explants display marked defects in their ability to generate vascular structures ( i , j , l , m ). Cell nuclei were stained with TOTO3 (blue). Scale bar, 100 μm. ( n ) Quantification of relative vessel length in the WT and Snail1 LOF explant cultures ( n =5 in each group). Data are presented as mean±s.e.m. ** P <0.01, Student’s t -test. Full size image Snail1 directs vessel patterning independent of vascular flow Given the global defects in vascular organization observed in Snail1 LOF embryos, we next considered the possibility that Snail1 may alter cardiac function with consequent (but indirect) effects on blood flow-induced vasculogenesis/angiogenesis [28] . As such, vascular remodelling was assessed ex vivo by isolating the allantois from E8.25 WT and Snail1 LOF littermates, and following their reorganization into vascular networks in explant cultures [29] . In the ex vivo system, cultured allantoises engage a vascularization programme similar, if not identical, to that observed in vivo with no requirements for vascular flow [29] . At pre-culture, allantois explants derived from Snail1 LOF mutants exhibit an immature vascular pattern similar to that observed in WT littermates ( Fig. 3h,k ). By contrast, at 24 h post culture, whereas WT explants readily undergo vascular morphogenesis while expressing Snail1 (as assessed in explants isolated from Snail1 LacZ/wt reporter mice) ( Fig. 3i,j and Supplementary Fig. 3g,h ), Snail1 LOF explants display an almost complete defect in their ability to organize into vascular networks ( Fig. 3i-n ). Under these conditions, no significant differences in TUNEL-positive ECs were observed between WT and Snail1 LOF mutant explant cultures ( Supplementary Fig. 3i ), highlighting the importance of Snail1 in supporting neovessel formation under flow-independent conditions. To further assess a vascular EC-specific role of Snail1 in controlling the angiogenic program in vivo , the ability of WT and Snail1 KO ECs to support neovessel formation in a transplant assay system was assessed [30] . To this end, ECs were isolated from β-actin-eGFP;Snail1 fl/fl mice and transduced with either a control Adeno-βgal or an Adeno-Cre construct in vitro and cultured alone or stimulated with VEGF ( Fig. 4a ). As shown in Fig. 4b , VEGF-stimulated ECs markedly increase Snail1 protein levels in Adeno-βgal-infected cells, but not in Adeno-Cre-expressing cells. Furthermore, when green fuorescent protein (GFP)-expressing control ECs are seeded into poly- L -lactic acid scaffolds and transplanted into recipient immunoincompetent hosts, neovessels are formed readily ( Fig. 4c,d ). As such, the ability of control and Snail1-deleted ECs to mount an angiogenic response in recipient mice was assessed in the absence or presence of exogenous VEGF. In the absence of VEGF, Adeno-βgal-transduced ECs form small networks of GFP + /PECAM-1 + vascular structures ( Fig. 4e,f ). By contrast, Snail1-deleted ECs are unable to organize into vascular networks ( Fig. 4g,h ). Following VEGF supplementation, Adeno-βgal-transduced ECs dramatically enhance their angiogenic potential, while Snail1-deleted ECs are unable to mount morphogenic responses despite the fact that these 2-week-old implants contain larger numbers of single ECs with no increase in apoptosis ( Fig. 4i and Supplementary Fig. 4 ). Taken together, these data support an EC-autonomous role for Snail1 in supporting the angiogenic programme. 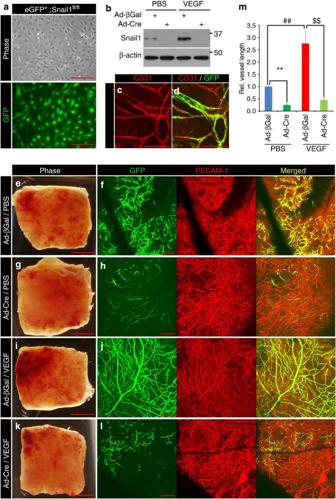Figure 4: Snail1 regulates angiogenic programme in a xenograft transplant model. (a) Representative image of isolated ECs from eGFP+;Snail1fl/flmice. Scale bar, 50 μm. (b) Adeno-β-gal or Adeno-Cre-infected ECs were stimulated with vehicle or VEGF (100 ng ml−1) for 12 h and subjected to western blot analysis. Results are representative of three or more experiments. (c,d) Whole-mount PECAM-1 (CD 31) staining of the implants after 14 din vivo. Scale bar, 50 μm. (e,g,i,k) Gross view of implants. Scale bar, 2 mm. (f,h,j,l) Whole-mount PECAM-1 staining of the implants. Scale bar, 100 μm. (m) Quantification of relative vessel length in the implants (n=3 in each group). Data are presented as mean±s.e.m. **,$$,##P<0.01, analysis of variance test. Figure 4: Snail1 regulates angiogenic programme in a xenograft transplant model. ( a ) Representative image of isolated ECs from eGFP + ;Snail1 fl/fl mice. Scale bar, 50 μm. ( b ) Adeno-β-gal or Adeno-Cre-infected ECs were stimulated with vehicle or VEGF (100 ng ml −1 ) for 12 h and subjected to western blot analysis. Results are representative of three or more experiments. ( c , d ) Whole-mount PECAM-1 (CD 31) staining of the implants after 14 d in vivo . Scale bar, 50 μm. ( e , g , i,k ) Gross view of implants. Scale bar, 2 mm. ( f , h , j , l ) Whole-mount PECAM-1 staining of the implants. Scale bar, 100 μm. ( m ) Quantification of relative vessel length in the implants ( n =3 in each group). Data are presented as mean±s.e.m. **, $$ , ## P <0.01, analysis of variance test. Full size image EC-specific deletion of Snail1 upregulates Notch signalling To assess the global impact of Snail1 expression on endothelial function in an unbiased fashion, primary ECs isolated from E10.5 Snail1 fl/fl embryos were transduced with either a control Adeno-β-gal or an Adeno-Cre construct in vitro , RNA isolated and subjected to transcriptional profiling. Remarkably, using a minimum of twofold change as a cutoff, Snail1 deletion alters the expression of ~500 unique transcripts with marked effects noted in gene ontologies associated with angiogenesis-associated functions ( Fig. 5a,b ). Unexpectedly, however, Snail1-KO ECs also display increased expression of multiple Notch targets, including Dll4 , Notch1 , Jag1 , Hey1 , guanylate cyclase 1 beta 3 ( GUCY1 β 3 ), meningiomal 1 ( MN1 ), insulin growth factor ( IGF2 ) and fibroblast growth factor 13 ( FGF13 ) [2] , [31] . Furthermore, arterial markers, including ephrin-B2 and Depp (also known as 8430408G22Rik [32] ), are also upregulated in Snail1 KO ECs, suggesting that the deletion of Snail1 may interface with arterial specification/differentiation ( Fig. 5c ). Validating the microarray data, quantitative reverse transcription–PCR (qRT–PCR) analyses confirm upregulated Notch-associated transcript levels in Snail1 KO ECs ( Fig. 5d ). Furthermore, when EC lysates are subjected to immunoblotting with specific antibodies directed against Dll4 or the intracellular domain of Notch1 (N1ICD), Snail1-KO ECs markedly increase protein levels of Dll4 and N1ICD relative to WT ECs ( Fig. 5e ). As these data were obtained from in vitro -cultured ECs wherein Snail1 was deleted after isolation, we sought to confirm the ability of Snail1 deletion to upregulate Dll4/Notch signalling in vivo . Hence, the status of Notch signalling-associated transcripts was assessed in ECs freshly isolated—and without in vitro culture—from E10.5 Snail1 LOF mutant and WT embryos. Consistent with the in vitro data, purified ECs from Snail1 LOF mutants display significantly higher levels of Dll4 , Notch1 , Hey1 and ephrin-B2 , confirming upregulated Notch signalling in the in vivo setting ( Fig. 5f ). In an effort to extend these observations to increases in protein expression levels in situ , tissue sections from E10.5 WT and Snail1 LOF mutants were immunostained for Dll4 and ephrin-B2. As predicted, both Dll4 and ephrin-B2 levels are markedly increased in the DA of Snail1 LOF mutant embryos (compare Fig. 5g,h,j,k and Fig. 5m,n,p,q ). Furthermore, Snail1 LOF ECs misexpress Dll4 and ephrin-B2 in cardinal vein fields ( Fig. 5h,i,k,l,n,o,q,r ). 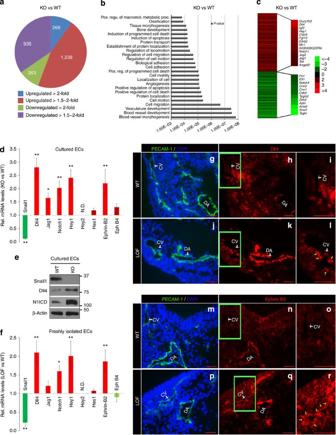Figure 5: Upregulated Notch signalling in Snail1-deleted ECs. (a–c) Transcriptional profiling analysis of cultured ECs derived from E10.5Snail1fl/flembryos and transducedin vitrowith Adeno-β-gal or Adeno-Cre to induce Snail1 KO recombination. Pie chart depicts the distribution of total transcripts changed in Snail1-deleted ECs as compared with control ECs (a). Gene ontology (GO) analysis of Snail1-deleted versus control ECs (b). Heat map representation of microarray data highlights the expression levels of key transcription factors, arterial–venous specification genes, EnMT-related genes, as well as Notch signalling target genes (c). (d) qRT-PCR analysis of cultured ECs froma. Snail1 KO ECs presented significantly higher levels ofDll4, Jag1,Notch1, Hey1andephrin-B2. Data are presented as mean±s.e.m. (n=3). *P<0.05, **P<0.01, Student’st-test. (e) Western blot analysis of cultured ECs froma. (f) qRT–PCR analysis of ECs freshly isolated from E10.5 WT and Snail1 KO embryos. ECs isolated from Snail1 LOF embryos displayed significantly higher levels ofDll4, Notch1, Hey1andephrin-B2(n=6 each). Data are presented as mean±s.e.m. *P<0.05, **P<0.01, Student’st-test. (g–l) Cross-sections from E10.5 WT and Snail1 LOF mutant embryos were co-stained with anti-PECAM-1 and anti-Dll4 antibodies. Cell nuclei were stained with DAPI (blue). (i,l) Magnified areas of boxed regions inhandk, respectively. Yellow arrow depicts Dll4-positive ECs in CV region. Scale bars, 50 μm. (m–r) Cross-sections from E10.5 WT and Snail1 LOF mutant embryos were co-stained with anti-PECAM-1 and anti-ephrin B2 antibodies. Cell nuclei were stained with DAPI (blue). (o,rmagnified areas of boxed regions innandq, respectively. Yellow arrows depict ephrin B2-positive ECs in CV region. Scale bars, 50 μm. Figure 5: Upregulated Notch signalling in Snail1-deleted ECs. ( a – c ) Transcriptional profiling analysis of cultured ECs derived from E10.5 Snail1 fl/fl embryos and transduced in vitro with Adeno-β-gal or Adeno-Cre to induce Snail1 KO recombination. Pie chart depicts the distribution of total transcripts changed in Snail1-deleted ECs as compared with control ECs ( a ). Gene ontology (GO) analysis of Snail1-deleted versus control ECs ( b ). Heat map representation of microarray data highlights the expression levels of key transcription factors, arterial–venous specification genes, EnMT-related genes, as well as Notch signalling target genes ( c ). ( d ) qRT-PCR analysis of cultured ECs from a . Snail1 KO ECs presented significantly higher levels of Dll4, Jag1 , Notch1, Hey1 and ephrin-B2 . Data are presented as mean±s.e.m. ( n =3). * P <0.05, ** P <0.01, Student’s t -test. ( e ) Western blot analysis of cultured ECs from a . ( f ) qRT–PCR analysis of ECs freshly isolated from E10.5 WT and Snail1 KO embryos. ECs isolated from Snail1 LOF embryos displayed significantly higher levels of Dll4, Notch1, Hey1 and ephrin-B2 ( n =6 each). Data are presented as mean±s.e.m. * P <0.05, ** P <0.01, Student’s t -test. ( g – l ) Cross-sections from E10.5 WT and Snail1 LOF mutant embryos were co-stained with anti-PECAM-1 and anti-Dll4 antibodies. Cell nuclei were stained with DAPI (blue). ( i , l ) Magnified areas of boxed regions in h and k , respectively. Yellow arrow depicts Dll4-positive ECs in CV region. Scale bars, 50 μm. ( m – r ) Cross-sections from E10.5 WT and Snail1 LOF mutant embryos were co-stained with anti-PECAM-1 and anti-ephrin B2 antibodies. Cell nuclei were stained with DAPI (blue). ( o , r magnified areas of boxed regions in n and q , respectively. Yellow arrows depict ephrin B2-positive ECs in CV region. Scale bars, 50 μm. Full size image Given that the phenotype and gene expression profile of Snail1 LOF mutant mice are consistent with exaggerated Dll4-Notch1 signalling [4] , [5] , [6] , we next tested the ability of the Notch signalling inhibitor, DAPT, to potentially rescue a portion of the vascular defects observed in the mutant mice [6] , [33] . To this end, timed pregnant mice were treated with a non-toxic, low dose of DAPT in an effort to decrease, but not totally inhibit, Notch signalling [6] , [33] . Confirming the efficacy of this treatment protocol, cross-sections and whole cell lysates recovered from DAPT-treated WT embryos display a marked reduction in N1ICD expression as assessed by N1ICD immunofluorescent staining and western blot analysis ( Supplementary Fig. 5a–g ). However, whereas partial inhibition of Notch signalling does not affect vascular patterning in WT embryos, DAPT-treated Snail1 LOF embryos display improved levels of vascular remodelling/branching in both the cephalic region ( Fig. 6a–d and Supplementary Fig. 6a,b ) and yolk sac ( Fig. 6e and Supplementary Fig. 6c–h ). Further, these changes occur in tandem with decreased Notch signalling in vivo as assessed by reduced Hey1 and ephrin-B2 expression ( Fig. 6f ). Although DAPT-treated Snail1 LOF embryos displayed a trend towards larger size, in a fashion consistent with improved vascular remodelling, the differences did not reach statistical significance ( Fig. 6g ). Importantly, increased vascular remodelling in Snail1-deleted cells is not confined to the in vivo setting and can be confirmed ex vivo in DAPT-treated explants of Snail1 LOF allantoises ( Fig. 6h–l ). Finally, to determine the impact of decreasing Notch signalling in ECs directly, WT or Snail1-deleted ECs were cultured atop Matrigel hydrogels in the absence or presence of DAPT in vitro [4] . Following Snail1 excision in Adeno-Cre-transduced Snail1 f/f ECs, sprouting behaviour is completely inhibited relative to Adenoβ-gal-transduced controls ( Supplementary Fig. 6i-l,q,r ). By contrast, in response to DAPT treatment, Snail1-deleted ECs decrease N1ICD expression to control levels and likewise recover a significant portion of their morphogenic activity ( Supplementary Fig. 6m-r ). 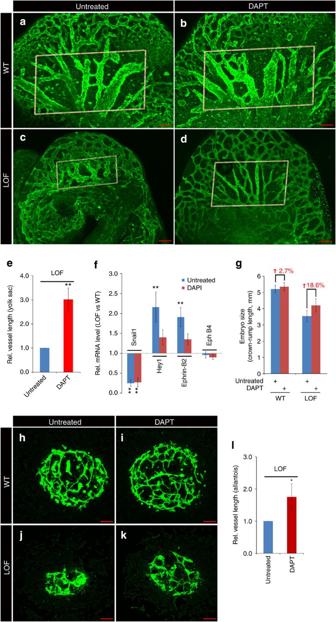Figure 6: Administration of DAPT partially reverses Snail1 deletion-induced vascular defects. Confocal analysis of PECAM-1 stained whole-mounted untreated (a,c) or DAPT-treated embryos (b,d). Rectangled area highlights improved vascular remodelling in DAPT-treated Snail1 LOF mutant embryos. Scale bar, 100 μm. (e) Quantification of relative vessel length in yolk sacs from E10.5 untreated and DAPT-treated Snail1 LOF embryos (n=4 each). Data are presented as mean±s.e.m. *P<0.05, **P<0.01, Student’st-test. (f) qRT–PCR analysis of ECs freshly isolated from untreated or DAPT-treated E10.5 embryos (n=4 each). Data are presented as mean±s.e.m. **P<0.01, Student’st-test. (g) Quantification of embryo size ina–dabove. Allantoises dissected from WT (h,i) and Snail1 LOF mutant (j,k) embryos were cultured in the presence of vehicle (h,j) or 8 μM DAPT (i,k) for 24 h and ECs visualized by whole-mount PECAM-1 staining. Scale bar, 100 μm. (l) Quantification of relative vessel length in allantoises (n=4 each). Data are presented as a mean±s.e.m. **P<0.05, Student’st-test. Figure 6: Administration of DAPT partially reverses Snail1 deletion-induced vascular defects. Confocal analysis of PECAM-1 stained whole-mounted untreated ( a , c ) or DAPT-treated embryos ( b , d ). Rectangled area highlights improved vascular remodelling in DAPT-treated Snail1 LOF mutant embryos. Scale bar, 100 μm. ( e ) Quantification of relative vessel length in yolk sacs from E10.5 untreated and DAPT-treated Snail1 LOF embryos ( n =4 each). Data are presented as mean±s.e.m. * P <0.05, ** P <0.01, Student’s t -test. ( f ) qRT–PCR analysis of ECs freshly isolated from untreated or DAPT-treated E10.5 embryos ( n =4 each). Data are presented as mean±s.e.m. ** P <0.01, Student’s t -test. ( g ) Quantification of embryo size in a – d above. Allantoises dissected from WT ( h , i ) and Snail1 LOF mutant ( j , k ) embryos were cultured in the presence of vehicle ( h , j ) or 8 μM DAPT ( i , k ) for 24 h and ECs visualized by whole-mount PECAM-1 staining. Scale bar, 100 μm. ( l ) Quantification of relative vessel length in allantoises ( n =4 each). Data are presented as a mean±s.e.m. ** P <0.05, Student’s t -test. Full size image Snail1 directs transcriptional repression of Dll4 Early embryonic lethality, defective cranial and ISV formation, dysregulated expression of arterial markers and failures in the yolk sac remodelling of yolk SAC are all hallmarks in gain-of-function activation of the Notch1 signalling pathway, particularly the overexpression of Dll4 (refs 4 , 5 , 34 , 35 ). Given that Dll4 protein expression is enhanced in both the arterial and venous beds of Snail1 LOF mice ( Fig. 5 ), we next explored the possibility that Snail1 might regulate Dll4 expression directly. Snail1 exerts many of its transcriptional effects by binding to E-box elements (consensus sequence, CANNTG) within the promoter proximal region of target genes [13] . In this regard, initial searches identified multiple conserved E-box elements that are located within the proximal region of the murine Dll4 promoter (see below). Hence, 293T cells were transiently transfected with a reporter construct containing the luciferase gene under the control of full-length murine Dll4 promoter (that is, bp −3,631 to +76) [6] . Under these conditions, Dll4 promoter activity is efficiently repressed when co-transfected with a Snail1 expression vector relative to the control vector ( Supplementary Fig. 7a,b ). Similarly, overexpression of Snail1 in purified ECs significantly represses Dll4 promoter activity ( Fig. 7a ). To identify the minimal promoter element containing the essential regulatory regions, systematically deleted mutants of the Dll4 promoter region were constructed and the transcriptional activities of the mutants tested in purified WT ECs ( Fig. 7b ). The deletion of bp −2,027 to +76, bp −1,156 to +76 or bp −481 to +76 results in a loss of 98.5%, 97.3% or 83.2% of Dll4 promoter activity, respectively, suggesting that the bp −481 to +76 fragment serves as the Dll4 minimal promoter ( Fig. 7b ). To further define the E-box elements (at positions +43 to +48, −395 to −390 and −432 to −427) within this region, ECs were electroporated with reporter constructs harbouring successive point mutations in the 3 E-boxes (CANNTG → A ANNT A ). Snail1 expression dramatically decreases luciferase activity in the WT minimal promoter sequence, but not in the mutant construct ( Fig. 7c ). Conversely, although Snail1 KO ECs display a significantly increased luciferase activity when transduced with the WT minimal promoter sequence relative to WT ECs, the upregulated activity is lost in the presence of the mutant construct ( Fig. 7c,d ). After chromatin immunoprecipitation (ChIP) of FLAG-Snail1 in transfected ECs followed by quantitative PCR (qPCR) of the Dll4 promoter and upstream region, FLAG-Snail1 ChIPs are enriched in the P1 and P2 regions (containing E-box-1 and E-box-2/-3, respectively) of the Dll4 promoter, but not in the upstream P3 region, suggesting that Snail1 represses the transcriptional activity of Dll4 by specifically binding to these three E-box elements ( Fig. 7e ). As the ability of Snail1 to repress transcriptional activity of target genes has been linked to the recruitment of histone-modifying cofactors [36] , [37] , [38] , ChIP analyses in WT and Snail1-KO ECs were performed using antibodies directed against di- or trimethylated H3K4 (H3K4me2 or H3K4me3) and acetylated H3K9 (H3K9Ac), histone markers associated with increased transcriptional activity [36] , [37] , [38] . As shown in Fig. 7f , the levels of H3K4me2, H3K4me3 and H3K9Ac are significantly increased at the Dll4 promoter in Snail1 KO ECs relative to WT ECs. 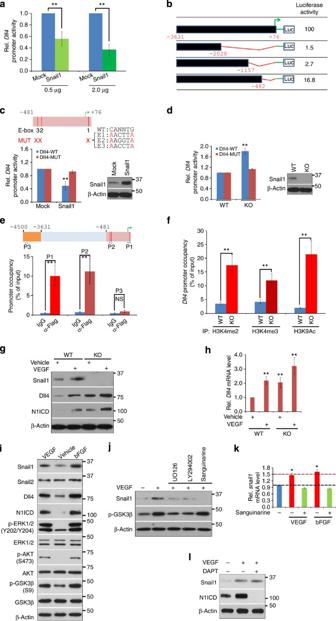Figure 7: EC Snail1 regulates Notch activity through direct transcriptional repression of Dll4. (a) ECs derived from E10.5 Snail1fl/flembryos were electroporated with a mock or Snail1 expression vector (0.5 or 2.0 μg) in combination with 0.5 μg of a mouseDll4promoter reporter construct and luciferase activity determined. (mean±s.e.m.;n=3). *P<0.05, **P<0.01, Student’st-test. (b) ECs fromawere electroporated with full-length or deletedDll4promoter reporter constructs and subjected to luciferase assay (results are of three experiments performed). (c) Diagram depicts the mutations in the three E-boxes located within the proximal region of the mouseDll4promoter. Cultured ECs fromawere electroporated with mock or human Snail1 expression vectors in combination with WT or mutated (MUT)Dll4promoter reporter constructs. Luciferase assays and western blot analysis are shown. (mean±s.e.m.;n=3). **P<0.01, Student’st-test. (d) Cultured control or Snail1-deleted ECs were electroporated with WT or MUTDll4promoter reporter constructs for luciferase assay (left) and western blot analysis (right). (mean±s.e.m.;n=3). **P<0.01, Student’st-test. (e) Snail1-Dll4promoter interactions in ECs expressing a Snail1 expression vector were assessed within the indicated regions (P1–P3) by ChIP/qPCR. (mean±s.e.m.;n=3). **P<0.01, Student’st-test. (f) Lysates from cultured control or Snail1-deleted ECs were subjected to ChIP analysis using antibodies directed against H3K4me2, H3K4me3 or H3K9Ac, andDll4occupancy determined by qPCR. (mean±s.e.m.;n=3). **P<0.01, Student’st-test. Control and Snail1-deleted ECs were treated with vehicle or VEGF for 12 h and subjected to western blotting (g) or qRT–PCR analysis (h), respectively. Western blotting results are representative of three experiments with qRT–PCR results presented as mean±s.e.m. (n=3). **P<0.01, analysis of variance (ANOVA). (i) WT ECs were stimulated with vehicle, VEGF (100 ng ml−1) or bFGF (20 ng ml−1) for 12 h and subjected to western blot analysis. Results are representative of three or more experiments. (j,k) WT ECs were pretreated with U0126 (20 μM), LY294002 (10 μM) or sanguinarine (2.5 μM) for 1 h followed by stimulation with VEGF or bFGF for 12 h. Cell lysates were prepared and subjected to western blotting (j) and qRT–PCR (k) analysis, respectively. Western blotting results representative of three experiments with qRT–PCR results presented as mean±s.e.m. (n=3). **P<0.01, ANOVA. (l) WT ECs were pretreated with vehicle or DAPT (8 μM) for 1 h followed by stimulation with VEGF (100 ng ml−1) for 12 h. Cell lysates were prepared and subjected to western blot analysis. Results are representative of three experiments. Figure 7: EC Snail1 regulates Notch activity through direct transcriptional repression of Dll4. ( a ) ECs derived from E10.5 Snail1 fl/fl embryos were electroporated with a mock or Snail1 expression vector (0.5 or 2.0 μg) in combination with 0.5 μg of a mouse Dll4 promoter reporter construct and luciferase activity determined. (mean±s.e.m. ; n =3). * P <0.05, ** P <0.01, Student’s t -test. ( b ) ECs from a were electroporated with full-length or deleted Dll4 promoter reporter constructs and subjected to luciferase assay (results are of three experiments performed). ( c ) Diagram depicts the mutations in the three E-boxes located within the proximal region of the mouse Dll4 promoter. Cultured ECs from a were electroporated with mock or human Snail1 expression vectors in combination with WT or mutated (MUT) Dll4 promoter reporter constructs. Luciferase assays and western blot analysis are shown. (mean±s.e.m. ; n =3). ** P <0.01, Student’s t -test. ( d ) Cultured control or Snail1-deleted ECs were electroporated with WT or MUT Dll4 promoter reporter constructs for luciferase assay (left) and western blot analysis (right). (mean±s.e.m. ; n =3). ** P <0.01, Student’s t -test. ( e ) Snail1- Dll4 promoter interactions in ECs expressing a Snail1 expression vector were assessed within the indicated regions (P1–P3) by ChIP/qPCR. (mean±s.e.m. ; n =3). ** P <0.01, Student’s t -test. ( f ) Lysates from cultured control or Snail1-deleted ECs were subjected to ChIP analysis using antibodies directed against H3K4me2, H3K4me3 or H3K9Ac, and Dll4 occupancy determined by qPCR. (mean±s.e.m. ; n =3). ** P <0.01, Student’s t -test. Control and Snail1-deleted ECs were treated with vehicle or VEGF for 12 h and subjected to western blotting ( g ) or qRT–PCR analysis ( h ), respectively. Western blotting results are representative of three experiments with qRT–PCR results presented as mean±s.e.m. ( n =3). ** P <0.01, analysis of variance (ANOVA). ( i ) WT ECs were stimulated with vehicle, VEGF (100 ng ml −1 ) or bFGF (20 ng ml −1 ) for 12 h and subjected to western blot analysis. Results are representative of three or more experiments. ( j , k ) WT ECs were pretreated with U0126 (20 μM), LY294002 (10 μM) or sanguinarine (2.5 μM) for 1 h followed by stimulation with VEGF or bFGF for 12 h. Cell lysates were prepared and subjected to western blotting ( j ) and qRT–PCR ( k ) analysis, respectively. Western blotting results representative of three experiments with qRT–PCR results presented as mean±s.e.m. ( n =3). ** P <0.01, ANOVA. ( l ) WT ECs were pretreated with vehicle or DAPT (8 μM) for 1 h followed by stimulation with VEGF (100 ng ml −1 ) for 12 h. Cell lysates were prepared and subjected to western blot analysis. Results are representative of three experiments. Full size image To address the ability of endogenously derived Snail1 to repress Dll4 expression and modulate Notch signalling, control or Snail1-deleted ECs were treated with VEGF, a potent agonist of Dll4 expression [7] , [8] , [39] . Under these conditions, VEGF-stimulated ECs increase Snail1 protein levels in tandem with increases in Dll4 and N1ICD expression ( Fig. 7g ). By contrast, in Snail1 KO ECs, Dll4 expression at both the mRNA and protein levels is enhanced in the absence of the endogenous Snail1-dependent feedback inhibition loop, resulting in increased levels of N1ICD ( Fig. 7h ). Recent studies have documented the ability of VEGF to trigger Snail1 expression in carcinoma cells [40] , [41] , but the mechanisms by which VEGF regulates Snail1 in ECs have not been characterized previously. VEGF-stimulated ECs are known to activate a series of signalling cascades, including ERK, phosphatidylinositol 3-kinase/Akt and nuclear factor- κB (NF-κB) [10] , [42] , [43] , that have each been implicated previously in regulating either Snail1 mRNA or protein expression [17] , [44] , [45] , [46] . Indeed, VEGF-dependent induction of Snail1, Dll4 and N1ICD, but not Snail2, in ECs occurs in tandem with the activating phosphorylation of ERK1/2 and Akt ( Fig. 7i ). Increased activation of ERK1/2 and Akt, in turn, triggers the Ser [9] phosphorylation/inactivation of glycogen synthase kinase 3β (GSK3β), the primary kinase responsible for Snail1 phosphorylation events that target the transcription factor for proteosomal destruction [17] , [38] , [45] ( Fig. 7i ). Similar, if not identical, results were observed with basic fibroblast growth factor (bFGF), a second pro-angiogenic growth factor that likewise increases Dll4 expression in ECs [47] ( Fig. 7i ). Finally, the central role played by GSK3β in Snail1 expression in ECs is confirmed by the ability of the synthetic GSK3 inhibitor, CHIR99021 (ref. 48 ), to directly increase EC Snail1 to near-maximal levels in the absence of either VEGF or bFGF ( Supplementary Fig. 7c ). To next determine the potential roles of ERK and/or Akt activation in controlling the GSK3β-dependent regulation of Snail1 protein levels, ECs were pretreated with the MEK/ERK inhibitor, UO126, or the phosphatidylinositol 3-kinase/Akt inhibitor, LY294002 (ref. 17 ). In the presence of either inhibitor, the VEGF- or bFGF- induced suppression of GSK3β activity is prevented, thereby blocking increases in Snail1 protein levels ( Fig. 7j and Supplementary Fig. 7d ). Furthermore, consistent with the ability of NF-κB to directly trigger Snail1 mRNA expression [44] , the specific NF-κB inhibitor, sanguinarine [46] , attenuates the VEGF- and bFGF-mediated upregulation of Snail1 mRNA and protein expression without affecting the VEGF-mediated suppression of GSK3β activity ( Fig. 7k and Supplementary Fig. 7d ). Although previous studies have reported the ability of Notch1 signalling itself to affect Snail1 expression [49] , [50] , Snail1 protein levels in VEGF-stimulated ECs are unaffected by DAPT despite an almost complete inhibition of N1ICD formation ( Fig. 7l ). Together, these observations describe a regulatory axis wherein VEGF triggers increased Snail1 mRNA expression in an NF-κB-dependent manner while stabilizing Snail1 protein via the ERK/Akt-dependent phosphorylation/ inactivation of GSK3β ( Fig. 8 ). 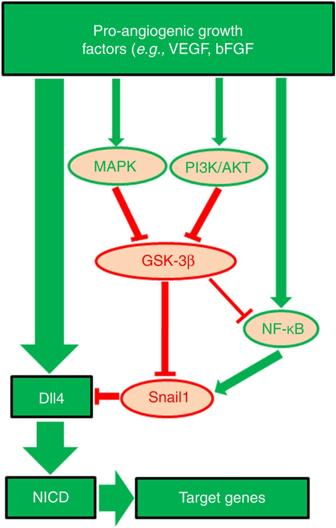Figure 8: Snail-dependent control of a Notch1-Dll4 regulatory cascade. Schematic outlining the ability of VEGF or bFGF to upregulate Dll4 expression and Notch signalling while simultaneously modulating Dll4 expression levels by co-inducing Snail1, resulting inDll4transcriptional repression. Figure 8: Snail-dependent control of a Notch1-Dll4 regulatory cascade. Schematic outlining the ability of VEGF or bFGF to upregulate Dll4 expression and Notch signalling while simultaneously modulating Dll4 expression levels by co-inducing Snail1, resulting in Dll4 transcriptional repression. Full size image Snail1 is most frequently characterized as a zinc-finger transcriptional repressor that triggers the EMT programmes critical to early embryogenesis [13] . Although the epiblast-specific conditional deletion of Snail1 leads to a series of complex cardiovascular network defects [15] , [16] , we now report that the conditional deletion of Snail1 in ECs leads to early embryonic lethality in association with profound alterations in vascular development. Although only a subset of ECs in the Snail1 LacZ/wt expressed β-galactosidase activity at the time points selected, these determinations do not allow for the tracking of Snail1 expression in a dynamic manner, as staining only reflects the steady state concentration of the enzyme at the time of assay. Alternatively, as observed during endothelial tip cell formation, changes in gene expression limited to small subsets of the developing vasculature can exert lethal effects during embryogenesis [1] , [2] , [3] . Future studies using Snail1 promoter-Cre transgenic lines and ROSA indicator strains should allow for a more rigorous lineage tracking of Snail1-expressing ECs during early development. Transcriptional profiling of WT versus Snail1-deleted ECs uncovered a surprisingly complex range of Snail1-regulated targets, but our attention was drawn to the significant increases in Notch1 signalling and Dll4 expression in combination with increased levels of downstream target genes [4] , [5] , [31] , [35] , [39] . Importantly, similar changes in the Notch-Dll4 signalling axis were confirmed both in vivo , in ECs isolated directly from Snail1 LOF mutant embryos and following Snail1 excision from floxed ECs in vitro . Furthermore, many of the vascular defects in vessel branching and remodelling observed in our Snail1 LOF mutants, including defects in the embryonic and extraembryonic vasculature, resemble those described in mouse embryos engineered to express constitutively active Notch1 or Notch4 as well as increased levels of N1ICD or Dll4 (refs 4 , 5 , 35 , 51 , 52 ). Given the fact that the range of Snail1 targets within the endothelium extends far beyond the Notch1/Dll4 signalling axis, it is unlikely that all of the Snail1 LOF mutant vascular phenotypes would be expected to duplicate precisely those observed in more targeted interventions designed to specifically upregulate Notch signalling. For example, whereas Dll4 or N1ICD overexpression frequently, but not always, increases artery diameter [4] , [5] , [35] , [47] , [52] , we did not note significant effects on artery size in our model. It should be stressed, however, that experimental systems designed to overexpress Notch/Notch ligands are far different from the model described herein where endogenous Snail1 was deleted, leading to more ‘physiologic’ compensatory increase in Notch signalling. Nevertheless, many of the vascular defects observed in Snail1 LOF mutant embryos were partially reversed following DAPT treatment in vivo , in allantois explants ex vivo and in isolated ECs cultured in vitro , underlining the importance of Notch1 signalling-related targets. Interestingly, the degree of rescue observed following treatment of Snail1 LOF mutant embryos with DAPT parallel closely with those observed in an EC-specific, β-catenin gain-of-function mutant mouse model that similarly displays enhanced Dll4 expression and an embryonic lethal phenotype [6] . Increases in Notch signalling in Snail1 LOF mutant embryos as well as isolated ECs are likely to be byproducts of the observed increases in both Notch1 and Dll4 expression. However, as increased levels of the Notch1 receptor alone (that is, in the absence of increased ligand expression or ligand-independent activation) are not predicted to drive, in and of themselves, robust N1ICD-dependent Notch signalling [53] , [54] , our attention turned to the effects of Snail1 on Dll4 expression as a potentially key effector of enhanced Notch signalling. Indeed, the Dll4 promoter was found to contain a series of E-boxes that serve as binding sites critical to Snail1 transcriptional repressor activity. Hence, in tandem with the VEGF-induced increase in Dll4 expression, VEGF also triggers Snail1 transcription and the post-translational stabilization of the protein via both GSK3β-independent (that is, NF-κB) and -dependent (that is, ERK/Akt) pathways. In turn, Snail1 fine-tunes Dll4 protein levels, and consequently, Notch1 activity, by serving as a transcriptional repressor of Dll4 expression. Although we have focused on the interplay between VEGF, Snail1 and Dll4 in regulating vascular behaviour, other signalling cascades are likely to be engaged in vivo , including the canonical Wnt pathway [6] , [9] . Of note, Wnt signalling also regulates Snail1 activity via GSK3β-dependent pathways [38] , [45] , raising the possibility that each of the multiple signalling transduction cascades interfacing with Dll4 expression and Notch activity also intersect with Snail1 as a negative feedback regulator. The ability of Snail1 to modulate Dll4 promoter expression, Dll4 mRNA or Dll4 protein levels in arterial beds, however, does not provide insights into the means by which Dll4 expression is inappropriately upregulated in the developing venous vasculature of the Snail1 LOF mutant mice. Recent studies have established that the 5′-promoter region of Dll4 does not serve to direct arterial versus venous patterns of expression [7] , [8] . Rather, the arterial EC-specific enhancer lies largely within the third Dll4 intron [7] , [8] . Interestingly, however, this intron contains an RBJK-binding site, and overexpression of N1ICD alone induces the Dll4-dependent arterialization of veins [8] , [34] . Indeed, Snail1 LOF mutant embryos also display increased levels of Dll4 and the N1ICD-dependent target genes, ephrin - B2 and Hey1 , suggesting that Snail1-dependent regulation of Dll4 expression extends beyond direct effects on the 5′-genomic region of Dll4 alone. In this regard, preliminary studies indicate that Snail1 also acts as a direct repressor of the Notch1 promoter ( Supplementary Fig. 8 ), raising the possibility that inappropriate Notch1 expression may participate in the misregulated expression of Dll4 in venous beds. The precise steps responsible for activating Notch1 in the venous beds of mutant mice require further study, but we note that Dll4 itself can exert long-distant effects following its release into exosomes and that ADAM 17 (upregulated more than twofold in Snail1 KO ECs; see deposited microarray data) can activate Notch1 signalling in a ligand-independent manner [54] , [55] . Notwithstanding the molecular details underlying this process, our data suggest that EC-derived Snail1 also plays an important role in controlling artery–vein specification during early development. As Snail1 LOF mice maintain the ability to assemble vascular plexus networks in both cranial fields and yolk sacs, major defects appear to arise in the vessel remodelling phase of development, a conclusion consistent with the observed defects in allantois explants and isolated ECs. Further studies will be required to determine the degree to which Snail1 drives vessel remodelling by affecting motile responses and artery–vein specification, as well as complementary processes critical to these events. Indeed, earlier studies for our laboratory have identified a role for Snail1 in regulating tissue-invasive programmes that are likely to participate in vessel morphogenesis [17] . The formation of a stable vasculature not only requires the induction of the necessary EC morphogenetic programmes, but also the recruitment of mural cell populations (that is, vascular smooth muscle cells or pericytes) to the abluminal wall of developing neovessels [56] . As such, we were intrigued by the fact that Snail1 LOF mutant embryos are unable to develop a mural cell coat. Similar observations have been observed following the upregulation of Notch1 activity in vivo [5] , [35] , and we considered the possibility that Snail1 induces an endothelial–mesenchymal transition (EnMT) programme that allows ECs themselves to serve as mural cell precursors. However, recent EC lineage tracking studies indicate that mural cells are recruited from the surrounding mesoderm rather than from the endothelium proper [57] . Indeed, although we were able to detect Snail1 expression in perivascular cell populations, mesoderm-specific Snail1 deletion did not have an impact on vascular development to the degree observed with EC-specific targeting. As such, Snail1 is more likely to control mural cell recruitment in trans through paracrine signalling pathways (for example, platelet-derived growth factor, transforming growth factor-β, Ang1/Tie2 or Notch signalling) [56] . Alhough Snail1-dependent EnMT programmes are unlikely engaged to generate mural cells during development, EC-like endocardial cells are known to express Snail1 and undergo a distinct phenotypic switch to mesenchymal-like cells in the developing cardiac cushions [2] , [50] , [58] . Nevertheless, the role of Snail1 in this process remains controversial with earlier reports debating its potential importance relative to that of Snail2/Slug as the critical EnMT effector [50] , [58] , [59] . Although prior analyses of Tie2 -Cre-targeted Snail1 heterozygote mice revealed only subtle defects in cardiac cushion cellularization [60] , we have found that Snail1 LOF mutant mice are unable to activate the associated EnMT programme ( Supplementary Fig. 9 ). These findings serve to highlight the broader roles played by Snail1 in regulating endothelial as well as endocardial function in the developing vasculature and cardiac fields, respectively, and support a model wherein the embryonic lethal phenotype of Snail1 LOF mice arises as a consequence of multiple defects in cardiovascular development. Broader roles for the Snail1-dependent regulation of EC function may extend into the postnatal setting as well. In preliminary studies, we have attempted to delete Snail1 postnatally to determine its role in retinal development ( Supplementary Fig. 10 ). Despite deleting Snail1 by ~70%, defects in retinal angiogenesis were not detected ( Supplementary Fig. 10 ) and additional studies are underway to delete Snail1 with higher efficiency to rule out the rescue of vascular responses by ECs that escaped Cre-mediated excision. This caveat aside, we find that Snail1-deleted ECs are unable to support the wound-like angiogenic responses that occur following transplantation into adult mice. Indeed, Snail1 has been detected in the neovasculature surrounding human carcinomas, raising the possibility that Snail1–Dll4 interactions direct vascular remodelling, and possibly lymphangiogenesis, in neoplastic states [61] , [62] , [63] , [64] . As adult ECs can also inappropriately re-activate embryonic programmes during pathologic fibrotic states to generate tissue fibroblasts [65] , a potential role for Snail1 in these postnatal events will be the subject of future studies. Mice Mice were housed under standard condition and protocols approved by the University Committee on Use and Care of Animals. Mice carrying Snail1 alleles [17] and mice with Snail1-LacZ knock-in alleles [23] were generated and maintained in our laboratory. Tie2 -Cre, Vav1 -Cre, Dermo1 -Cre and β-actin-GFP transgenic mice were obtained from Jackson Laboratory. VE-cadherin-Cre ERT2 transgenic mice were provided by ML Iruela-Arispe (University of California, Los Angeles) [66] . Littermate controls of both sexes were used in all experiments. All mouse strains were backcrossed into the C57BL/6J background for at least seven generations. To inhibit Notch signalling in vivo , timed pregnant mice were injected subcutaneously with 100 mg kg −1 DAPT (Tocris Bioscience) dissolved in 10% ethanol and 90% corn oil at E7.5, E8.5 and E9.5 with the embryos dissected at E10.5 (ref. 6 ). Gene inactivation in Snail1 LacZ/fl ; VE-cadherin -Cre-ERT2 + embryos was triggered by intraperitoneal injections of 150 μl of tamoxifen solution (10 mg ml −1 , dissolved in 1:10 ethanol/corn oil; Sigma) into pregnant females at E11.5 and E13.5. Gene inactivation in pups was triggered by intraperitoneal injections of 50 μl tamoxifen solution (10 mg ml −1 ) at P1 and P3. Eyes were retrieved from pups at P6 and fixed in 4% paraformaldehyde–PBS overnight at 4 °C. Retinas were dissected and subjected to whole-mount PECAM-1. Haematopoietic colony-forming assay For haematopoietic colony-forming assays, yolk sacs were isolated and incubated with 0.1% Collagenase D (Roche) in Hank’s PBS containing 10% FCS and Pen/Strep for 1 h at 37 °C with occasional agitation to aid dispersion of the tissue [67] . The cells were then washed and counted. For colony-forming unit (CFU) assays, 1.5 × 10 4 cells were seeded into 1 ml of methocellulose media supplemented with interleukin 3, interleukin 6 and stem cell factor (M3434, Stem Cell Technologies). Clones (>30 cells) were scored as myeloid (CFU-C) or erythroid (BFU-E) at day 7 of culture. Allantois explant culture Allantoises were dissected from E8.25 mouse embryos and placed individually on gelatin-coated chamber wells as described [16] . Explants were cultured in DMEM medium containing 15% fibronectin-depleted fetal bovine serum for 24 h. In selected experiments, allantois explants were cultured in vitro in the presence of 8 μM DAPT [6] . Pre-cultured or post-cultured explants were fixed in 4% paraformaldehyde–PBS and subjected to anti-PECAM-1 immunofluorescence or TUNEL assay. Immunofluorescence staining Embryos or yolk sacs were fixed in 4% paraformaldehyde–PBS for 2 h, permeabilized in 100% methanol for 30 min at −20 °C and incubated in blocking buffer (5% goat serum in PBS) containing anti-PECAM-1 primary antibody (1:500, BD Biosciences) overnight at 4 °C, followed by incubation with secondary antibodies (1:400, Alexa-Fluor-488-labelled, Invitrogen) in blocking buffer for 2 h. For frozen sections, allantois explant cultures or ECs, tissues/cells were fixed in 4% paraformaldehyde–PBS, permeabilized in PBST (PBS plus 0.3% Triton X-100) and incubated in blocking buffer (5% goat or donkey serum plus 2% BSA in PBS) with primary antibodies directed against PECAM-1 (1:500), α-SMA (1:500, Abcam), Dll4 or ephrin-B2 (1:200, R&D Systems), followed by incubation with secondary antibodies (1:400, Invitrogen). All images were processed using Image J and Photoshop CS5. Relative vascular density, vessel length and branch points were determined in multiple fixed areas of view in three or more WT versus LOF embryos, yolk sacs, allantois explants or EC xenografts as described [68] , [69] . EC isolation and culture EC isolation was performed as described previously with modifications [70] . Briefly, E10.5 Snail1 fl/fl embryos (of either male or female sex) or adult lungs (isolated from female mice) were dissected in ice-cold PBS and digested in a mixture of collagenase type I (Worthington), DNase I (Sigma-Aldrich) and dispase (Invitrogen) for 30 min at 37 °C. ECs were then separated using Dynabeads (Invitrogen) coated with anti-PECAM-1 antibody and cultured in DMEM medium supplemented with 20% fetal bovine serum (Invitrogen) and EC growth supplement (BD Biosciences). Confluent ECs were trypsinized and separated using Dynabeads coated with anti-ICAM-1 antibody (BD Biosciences). Following two rounds of sorting, the purity of ECs is ~90% and the cells were used within two passages of their initial isolation. To obtain Snail1 WT and KO ECs, cells were infected with adenoviral-βGal or adenoviral-Cre (MOI, 50), respectively. For in vitro assessments of EC morphogenesis, Snail1 WT and KO ECs were cultured atop Matrigel-coated dishes (BD Biosciences) in the absence or presence of DAPT (8 μm) for 12 h and imaged [4] . In selected experiments, ECs were freshly isolated from E10.5 WT and Snail1 LOF embryos using Dynabeads coated with anti-PECAM1 antibody, and subjected to microarray gene expression and qRT–PCR analyses. Angiogenic xenotransplant assay Angiogenic xenotransplant assays were performed as described previously with modifications [30] . In brief, cultured ECs derived from lungs of 1-month-old Snail1 fl/fl /β-Actin-GFP + mice were transduced in vitro with Adeno-Cre or Adeno-β-gal expression vectors. The recovered WT and Snail1-KO ECs were re-suspended in a 1:1 Matrigel mixture in the presence of PBS or 100 ng ml −1 VEGF-165 (R&D Systems) and absorbed into poly- L -lactic acid scaffolds (1 × 10 6 ECs each). The matrix implants were transplanted subcutaneously into male SCID mice, retrieved 14 days after implantation and imaged by phase-contrast microscopy, GFP fluorescence and whole-mount PECAM-1 immunofluorescent staining. Microarray gene expression assay and qRT–PCR Cultured WT, Snail1 fl/fl , Snail1-deleted or Snail1 KO embryonic ECs were isolated as described previously with modifications [70] . Total RNA was isolated with the RNeasy Mini Kit (Qiagen), labelled and then hybridized to Mouse 430 2.0 complementary DNA microarrays (Affymetrix). Differentially expressed probe sets were determined by using a minimum fold change of 1.5 in Snail1-deleted ECs relative to Snail1 fl/fl control ECs as described previously [48] . For qRT–PCR analysis, 0.5 μg total RNA was reverse transcribed into cDNA using SuperScript III cDNA Synthesis Kit (Invitrogen). cDNA was amplified using SYBR Green PCR mix (Applied Biosystems) and qPCR was carried out using an ABI PRISM 7900HT (Applied Biosystems) sequence detection system. For all samples, the expression level, normalized to the housekeeping gene encoding glyceraldehyde 3-phosphate dehydrogenase, was determined with the comparative threshold cycle (Ct) method (primers are listed in Supplementary Table 1 ). Immunoblot and ChIP assays Cultured WT and Snail1 KO ECs were stimulated with recombinant VEGF-A/164 (100 ng ml −1 ) or bFGF (20 ng ml −1 ) (both from R&D Systems), and the cell lysates were subjected to immunoblot assay using antibodies against Snail1 (1:1,000), Snail2 (1:1,000), N1ICD (1:1,000), p-ERK1/2 (Y202/204) (1:1,000), p-Akt (S473) (1:500), p-GSK3β (S9) (1:2,000), GSK3β (1:5,000), β-actin (1:10,000) (all from Cell Signaling), Dll4 (1:1,000) or α-SMA (1:5,000) (both from Abcam). For ChIP analysis, ECs were electroporated with FLAG-Snail1-expressing vector using Amaxa Basic Nucleofector kit (Lonza) and subjected to ChIP assay as described previously [38] . Luciferase reporter assay A 3.7-kb fragment of the mouse Dll4 promoter (−3,631 to +76) subcloned in the pGL3 basic vector was kindly provided by T. Kume (Northwestern University, Chicago, IL). The minimal Dll4 promoter (−481 to +76) was amplified from the 3.7-kb fragment of Dll4 promoter and subcloned in the pGL3 basic vector (Promega). The Dll4-MUT was generated by mutating the Snail1 binding sites (E-boxes) CANNTG to A ANNT A using the QuikChange Site-Directed Mutagenesis kit (Stratagene). A 1.2-kb fragment of the mouse Notch1 promoter (−1,039 to +182) was obtained from GeneCopoeia, Inc. Dual-luciferase reporter assays were performed according to the manufacturer’s instructions (Promega). Statistical analysis Statistical analysis was performed with the Student’s t -test or by analysis of variance. * P <0.05, ** P <0.01, $$ P <0.01, ## P <0.01. All experiments were repeated three or more times. How to cite this article: Wu, Z.-Q. et al . A Snail1/Notch1 signalling axis controls embryonic vascular development. Nat. Commun. 5:3998 doi: 10.1038/ncomms4998 (2014). Accession codes : Microarray data has been deposited in GEO under accession number GSE57030 .